Electron transfer and coupling in graphene–tungsten disulfide van der Waals heterostructures The newly discovered two-dimensional materials can be used to form atomically thin and sharp van der Waals heterostructures with nearly perfect interface qualities, which can transform the science and technology of semiconductor heterostructures. Owing to the weak van der Waals interlayer coupling, the electronic states of participating materials remain largely unchanged. Hence, emergent properties of these structures rely on two key elements: electron transfer across the interface and interlayer coupling. Here we show, using graphene–tungsten disulfide heterostructures as an example, evidence of ultrafast and highly efficient interlayer electron transfer and strong interlayer coupling and control. We find that photocarriers injected in tungsten disulfide transfer to graphene in 1 ps and with near-unity efficiency. We also demonstrate that optical properties of tungsten disulfide can be effectively tuned by carriers in graphene. These findings illustrate basic processes required for using van der Waals heterostructures in electronics and photonics. Forming heterostructures has been a key concept in solid-state science and an important tool to engineer the electronic and optical properties of semiconductors. Heterostructures formed by conventional semiconductors have led to important discoveries of integer [1] , fractional [2] and quantum spin Hall effects [3] , [4] , exciton–polariton condensations [5] and Bloch oscillations of electrons [6] . They are also basic building blocks for advanced technologies such as lasers and transistors [7] . However, owing to the lattice-matching conditions required by the epitaxial growth, the lattice constants and crystal structures of the involved materials must be similar. This severely limits the selection of materials and the quality of the interfaces. The newly developed monolayer two-dimensional crystals, such as graphene [8] , [9] , boron nitride [10] and transition metal dichalcogenides (TMDs) [11] , provide a new way to develop heterostructures and can potentially transform the science and technology of semiconductor heterostructures [12] . Since these heterostructures utilize the van der Waals interlayer interaction, lattice matching is no longer a significant factor. Hence, a large number of materials can be selected to form heterostructures. The interface is atomically sharp and the junction can be as thin as two atomic layers—both reaching the ultimate limits. A number of drawbacks in conventional heterostructures are in principle reduced in these van der Waals heterostructures, such as interfacial defects, interlayer atomic diffusion, strain and disorders. In addition, these structures are flexible and chemically stable. Their fabrication is compatible with current thin-film technologies. Since 2012, several groups have reported experimental studies of van der Waals heterostructures, most of which combined graphene with a multilayer TMD. For example, using TMD thin layers as tunnelling barriers and graphene as one or both electrodes, vertical tunnelling transistors with high on–off ratios and large current densities were demonstrated [13] , [14] , [15] , [16] . Photovoltaic devices using TMD as light absorption and graphene as charge-transfer components achieved promising efficiencies [17] , [18] . Owing to the weak van der Waals coupling, the electronic structures of the individual materials that form the heterostructure remain largely unchanged [19] , [20] , [21] . Hence, two important elements for such heterostructures are efficient electron transfer across the interface and control of one layer from the other via various interlayer-coupling mechanisms. First, in order to utilize the superior light-absorption properties of TMD and charge transport performance of graphene in photovoltaic devices, photocarriers generated in TMD must efficiently transfer to graphene before they recombine [22] . Controllable charge transfer is also a requirement for vertical transistors [22] , [23] . Second, coupling of electronic states between two layers allows control of one layer via the other, which is important for logic devices and modulators. As one example, Coulomb drag between two graphene layers separated by a thin insulating layer has been observed [24] , [25] , [26] . In the following, we use ultrafast spectroscopy to time-resolve the charge-transfer process from WS 2 to graphene. We find that photocarriers injected in monolayer WS 2 transfer to graphene in ~1 ps and with a near-unity efficiency. Efficient and ultrafast transfer of electron-hole pairs and excitons from bulk WS 2 to graphene is also observed. Furthermore, we find that carriers in graphene can significantly change the exciton resonance in monolayer WS 2 , which can be utilized in integrated optoelectronic devices with a gate-controllable optical response. Heterostructures of graphene–WS 2 monolayer We first study a WS 2 monolayer flake fabricated by mechanical exfoliation (see Method). In our pump–probe set-up, a 390-nm and 100-fs laser pulse with a peak fluence of 1 μJ cm −2 excites electron–hole pairs in the sample with a peak density of ~3.3 × 10 11 cm −2 , estimated by using an absorption coefficient [27] , [28] of 2.3 × 10 8 m −1 . To monitor the carrier and exciton dynamics, time-resolved differential reflection (Δ R / R 0 ) of a 620-nm probe pulse is measured. The differential reflection is defined as the pump-induced relative change of the probe reflection (see Method). As shown in Fig. 1a , the signal decays bi-exponentially (red line). The fast time constant of 1.3 ps could be associated with the exciton-formation process. If the injected electron–hole pairs can induce a differential reflection signal through screening effect, it can be larger than the effect of excitons. In this scenario, the signal would decrease as the electron–hole pairs form excitons. We note that such a fast component has also been observed in MoS 2 monolayers [29] , [30] , [31] . We attribute the slow time constant of 21 ps to the exciton recombination lifetime. The measurement is repeated with different probe wavelengths, and similar dynamics are observed. Symbols in Fig. 1e illustrate the probe-wavelength dependence of the peak signal. By comparing with the photoluminescence (PL) spectrum of the sample (the blue curve), we find that the line shape of the differential reflection signal is strongly correlated to, but different from, the exciton line shape. It has both positive and negative spectral regions, indicating rather complex mechanisms that induce the differential reflection. Similarly, complex transient absorption spectra have been observed in other TMD monolayers, such as MoS 2 (refs 30 , 32 ). Although further investigations are necessary to fully understand the mechanisms responsible for such line shapes, it is clear that the differential reflection originates from the exciton resonance, instead of other processes such as free-carrier absorption. 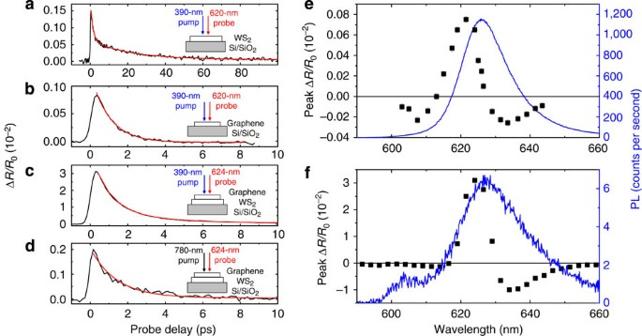Figure 1: Photocarrier dynamics in WS2monolayer, graphene and their heterostructures. (a) Differential reflection (ΔR/R0) measured from a monolayer WS2flake with a 390-nm pump and a 620-nm probe pulse. The red line indicates a biexponential fit with time constants of 1.3 and 21 ps. (b) The same measurement as (a) performed with a monolayer graphene sample. The red line is a single-exponential fit of 1 ps. (c) The same measurement as (a) performed with a heterostructure sample of graphene and monolayer WS2, and with a 624-nm probe pulse. The signal decays biexponentially with time constants of 1 and 3.5 ps. (d) The same measurement ascbut with a 780-nm pump pulse. The red line indicates a 1.4-ps exponential decay. (e) Peak differential reflection from the monolayer WS2as a function of the probe wavelength (symbols, left axis) and PL of the same sample under 405-nm laser excitation. The error bars indicate the uncertainties due to noise. (f) Same asebut for the heterostructure sample. Figure 1: Photocarrier dynamics in WS 2 monolayer, graphene and their heterostructures. ( a ) Differential reflection (Δ R / R 0 ) measured from a monolayer WS 2 flake with a 390-nm pump and a 620-nm probe pulse. The red line indicates a biexponential fit with time constants of 1.3 and 21 ps. ( b ) The same measurement as ( a ) performed with a monolayer graphene sample. The red line is a single-exponential fit of 1 ps. ( c ) The same measurement as ( a ) performed with a heterostructure sample of graphene and monolayer WS 2 , and with a 624-nm probe pulse. The signal decays biexponentially with time constants of 1 and 3.5 ps. ( d ) The same measurement as c but with a 780-nm pump pulse. The red line indicates a 1.4-ps exponential decay. ( e ) Peak differential reflection from the monolayer WS 2 as a function of the probe wavelength (symbols, left axis) and PL of the same sample under 405-nm laser excitation. The error bars indicate the uncertainties due to noise. ( f ) Same as e but for the heterostructure sample. Full size image Under the same conditions, we measure a monolayer graphene sample, as shown in Fig. 1b . Here the 390-nm pump excites a peak carrier density of 5 × 10 10 cm −2 . The single-exponential decay (red curve) with a time constant of 1 ps indicates the ultrashort carrier lifetime in graphene. Having investigated the two components individually, we now perform the same measurement with a graphene–WS 2 heterostructure sample, which was made by putting an exfoliated graphene flake on top of a monolayer WS 2 flake. The 390-nm pump pulse excites electron–hole pairs in both layers with densities similar to the first two measurements. The differential reflection of a 624-nm probe is shown in Fig. 1c . We see two astonishing features. First, the magnitude of the signal is 20 and 30 times higher than the individual WS 2 and graphene samples, respectively. The signal is proportional to the pump fluence ( Supplementary Fig. 1 ). Second, the decay of the signal is much faster than WS 2 , described by two time constants of 1 and 3.5 ps. Similar to the individual WS 2 sample, we find that the differential reflection depends strongly on the probe wavelength, as shown in Fig. 1f (see also Supplementary Fig. 2 ). Hence, the exciton resonance of WS 2 is responsible for the differential reflection signal. However, electron–hole pairs and excitons in WS 2 at this density level do not induce such a large signal, and do not decay in a few picoseconds ( Fig. 1a ). Hence, both the magnitude and the decay time of the signal indicate that the excitonic resonance in WS 2 is changed by the presence of carriers in graphene. To further confirm such an interlayer coupling, we use a 780-nm pump pulse with a fluence of 0.2 μJ cm −2 to selectively inject carriers in the graphene layer, with a density of 2 × 10 10 cm −2 . The WS 2 layer is not excited, since the pump photon energy is not sufficient for one-photon absorption, while its intensity is too low for two-photon absorption to inject a significant carrier density. The differential reflection of the 624-nm probe is observed, as shown in Fig. 1d and Supplementary Fig. 3 . The same measurement performed with the individual WS 2 monolayer and graphene samples yielded no detectable signal, further confirming that the WS 2 layer in the heterostructure is not excited by the 780-nm pump. These measurements prove that carriers in graphene cause a change of the exciton resonance in WS 2 . In an individual TMD monolayer, a significant amount of electric field lines between holes and electrons extends to the vacuum surrounding the monolayer. Hence, the screening of the field is greatly suppressed, resulting in an unusually strong Coulomb interaction between electrons and holes, and a large exciton-binding energy. When the TMD monolayer forms a heterostructure with a graphene layer, carriers in graphene effectively screen the field, and hence alter the exciton resonance of the TMD. On the basis of our results, the screening effect of carriers in graphene is much stronger than those in WS 2 . We attribute this to the much higher mobility of carriers in graphene compared with TMDs. This effect suggests the possibility of controlling optical properties of TMDs via gate control of carrier density in graphene in such heterostructures. However, further measurements with gate control are necessary to study the feasibility of this approach. The results summarized in Fig. 1 also provide unambiguous evidence of ultrafast and efficient transfer of photocarriers from WS 2 to graphene. First, since carriers with a density of 2 × 10 10 cm −2 give rise to a signal of 2 × 10 −3 ( Fig. 1d ), the signal of 0.03 induced by the 390-nm pump ( Fig. 1c ) corresponds to a carrier density in graphene of 3 × 10 11 cm −2 . This is reasonably consistent with the total carrier density injected in the heterostructure by the 390-nm pump. Hence, carriers injected in WS 2 must rapidly transfer to graphene in order to cause the signal. Second, the fast decay of the signal shown in Fig. 1c indicates that most carriers in WS 2 transfer to graphene on a picosecond timescale, and then recombine in graphene rapidly. Otherwise, one would expect a slow decay on the order of 20 ps, as measured in Fig. 1a . Third, the PL from the heterostructure sample is ~170 times weaker than the individual WS 2 sample, as shown in Fig. 1e,f . Such a significant quenching effect of graphene indicates that in the heterostructure sample, nearly 100% of the carriers excited in WS 2 transfer to graphene, instead of recombining in WS 2 . Heterostructures of graphene–WS 2 bulk We next extend these measurements to a heterostructure formed by graphene and bulk WS 2 , partially motivated by the fact that most recent studies of graphene-related heterostructures involved bulk-like TMD layers [13] , [14] , [15] , [16] , [17] , [18] . We first excite a region of a thick WS 2 flake that is not covered by graphene with a 390-nm and 1 μJ cm −2 pump pulse. The thickness of this flake is in the range of 25–30 nm. It can be treated as a bulk sample. The differential reflection of a 624-nm probe is shown as the blue circles in Fig. 2a and inset of Fig. 2b , for two time ranges. The signal decays biexponentially with time constants of 1.7 and 78 ps. We attribute the slow component to exciton lifetime in bulk WS 2 . It is about four times longer than the monolayer because of the suppressed recombination by its indirect bandgap. We repeat the measurement on a region of this flake that is covered by graphene. As shown as the black squares in Fig. 2 , the signal is slightly larger and decays faster (~50 ps, after an initial fast process of 1.5 ps). By repeating these measurements with different probe wavelengths, shown in Fig. 2b , we find that in both regions the differential reflection signals originate from the exciton resonance in WS 2 . 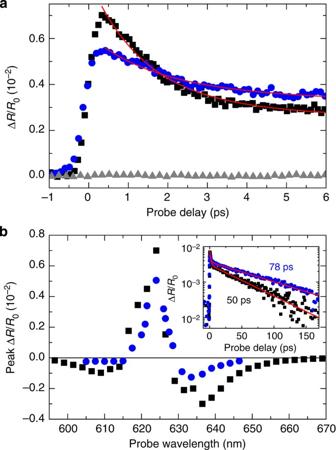Figure 2: Photocarrier dynamics in bulk WS2and its heterostructure with graphene. (a) Differential reflection (ΔR/R0) measured from a bulk WS2flake (blue circles) and a bulk WS2–graphene heterostructure (black squares) with a 390-nm pump and a 624-nm probe pulse. Inset ofbshows these signal over a longer time range. The grey triangles inaare measured from the heterostructure sample, but with a pump pulse of 780 nm. (b) Peak differential reflection signal as a function of the probe wavelength from the bulk WS2(blue circles) and the heterostructure (black squares) samples. Figure 2: Photocarrier dynamics in bulk WS 2 and its heterostructure with graphene. ( a ) Differential reflection (Δ R / R 0 ) measured from a bulk WS 2 flake (blue circles) and a bulk WS 2 –graphene heterostructure (black squares) with a 390-nm pump and a 624-nm probe pulse. Inset of b shows these signal over a longer time range. The grey triangles in a are measured from the heterostructure sample, but with a pump pulse of 780 nm. ( b ) Peak differential reflection signal as a function of the probe wavelength from the bulk WS 2 (blue circles) and the heterostructure (black squares) samples. Full size image On the basis of the absorption coefficient of bulk WS 2 , the pump and probe pulses penetrate ~10–20 atomic layers of WS 2 . Hence, electron–hole pairs are injected in these layers as well as in the graphene layer. Since the signal from both regions are comparable, the strong effect of carriers in graphene on WS 2 exciton resonance observed in graphene-monolayer WS 2 heterostructure is absent. To further confirm this, we use a 780-nm pulse of the same fluence to inject carrier in graphene only. No differential reflection signal was observed, as indicated as the triangles in Fig. 2a . The absence of this interlayer effect in bulk suggests that the effect is short-ranged or relies on the direct bandstructure of monolayers. However, the reduced exciton lifetime in the heterostructure, compared with the individual bulk WS 2 , provides additional evidence of efficient electron transfer from WS 2 to graphene, which serves as a fast decay channel. The slower dynamics, compared with the graphene-monolayer WS 2 heterostructure, can be attributed to the slow interlayer diffusion process of excitons in bulk WS 2 , which is necessary for these excitons to reach the junction. Finally, we study the electron transfer process from bulk WS 2 to graphene in a more direct manner, by selectively pumping the WS 2 layer and probing the graphene layer. A 620-nm pulse is used to resonantly inject excitons in bulk WS 2 . A 780-nm pulse is used to probe carriers in graphene that are transferred from WS 2 , as shown in Fig. 3 . Since the probe is below the exciton resonance of WS 2 , it does not probe WS 2 . To confirm this, we repeat the measurement in a region that is not covered by graphene, and observe no signal (blue circles in the inset of Fig. 3 ). Although the 620-nm pulse also injects carriers in graphene, they decay rapidly in 1 ps, which is further confirmed by repeating the measurement with an individual graphene sample (pink triangles). Hence, the long-lived signal from the heterostructure sample originates from excitons injected in WS 2 and then subsequently transferred to graphene. In this process, the WS 2 with a long exciton lifetime serves as a quasi-steady supply of carriers in graphene. The decay time of 69 ps (red line) is shorter than the exciton lifetime in bulk WS 2 , since both recombination in WS 2 and transfer to graphene contribute to the overall decay of exciton density. Furthermore, we note that unlike the 390-nm pump used earlier, the 620-nm pulse resonantly inject excitons, instead of free carriers. Hence, this measurement directly demonstrates transfer of excitons across the van der Waals heterostructure. 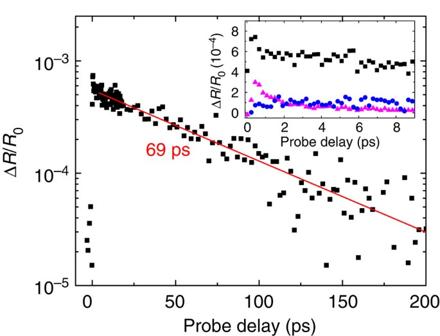Figure 3: Differential reflection measured from the bulk WS2–graphene heterostructure sample. The pump and probe wavelengths are 620 and 780 nm, respectively. The inset shows the same data near zero delay (squares) and those measured from individual graphene (pink triangles) and a bulk WS2(blue circles). Figure 3: Differential reflection measured from the bulk WS 2 –graphene heterostructure sample. The pump and probe wavelengths are 620 and 780 nm, respectively. The inset shows the same data near zero delay (squares) and those measured from individual graphene (pink triangles) and a bulk WS 2 (blue circles). Full size image We find that in van der Waals heterostructures formed by graphene and monolayer WS 2 , photocarriers injected in WS 2 transfer to graphene in ~1 ps and with a near-unity efficiency. Efficient and ultrafast transfer of electron–hole pairs and excitons are also observed in heterostructures of bulk WS 2 and graphene. Such fast and efficient excitation transfer processes are essential for applications in photovoltaics and photodetectors. We also found that carriers in graphene significantly change the exciton resonance in the WS 2 monolayer. A 3% change of the exciton absorption is induced by a rather moderate carrier density of 4 × 10 11 cm −2 . This can be utilized in integrated optoelectronic devices with a gate-controllable optical response, and provides a new and more efficient way to probe carrier dynamics in graphene. Sample fabrication High-quality WS 2 flakes were mechanically exfoliated from bulk synthetic WS 2 crystals on a SiO 2 (90 nm)/Si substrate. Monolayer flakes were identified by their optical contrast and later confirmed by PL measurements ( Fig. 1e ). The sample was cleaned with acetone and isopropanol and dried under nitrogen in order to remove the residue from the adhesive tape used for exfoliation. To prepare a graphene flake to be transferred, a SiO 2 /Si substrate was covered by a layer of polyvinyl alcohol and then a layer of poly(methyl methacrylate) (PMMA) [33] . Graphene flakes were mechanically exfoliated from bulk natural Kish graphite crystals on the PMMA layer. A monolayer graphene flake was identified by its optical contrast ( Supplementary Fig. 4 ) and later confirmed by its Raman spectrum ( Supplementary Fig. 5 ). The monolayer graphene flake is transferred on the WS 2 flake by using a micromanipulator with a microscope. After the transfer, the sample was cleaned with 1,2-Dichloroethane to remove polymer and tape residues. Finally, the sample was annealed at 250 °C for 2 h under H 2 -Ar (20-100 s.c.c.m.) environment at a base pressure of 3 Torr. A thick WS 2 flake close to the monolayer WS 2 flake is also partially covered by graphene ( Supplementary Fig. 4 ). The thickness of this flake is in the range of 25–30 nm, according to atomic force microscopy measurements ( Supplementary Fig. 6 ). Differential reflection measurements Since the substrates used for the samples are not transparent, transmission measurements are not feasible. Hence, we perform differential reflection measurements. In the differential reflection set-up, a 10-W solid-state diode laser is used to pump a passively mode-locked Ti:sapphire oscillator that generates 100-fs pulses with a central wavelength of 780 nm at 80 MHz. The majority of this beam (92%) is used to pump an optical parametric oscillator, which generates a signal output in the range of 1,100–1,500 nm. Second harmonic of this beam, in the range of 550–750 nm, is generated in a beta barium borate crystal. It provides one tunable beam for the measurements. The rest of the 780-nm beam is focused to another beta barium borate crystals to generate its second harmonic at 390 nm, used as another beam for the measurement. The 780-nm beam itself can also be used in the measurement. Depending on the purpose of each measurement, two of these three beams are selected. We measure differential reflection of the probe induced by the pump. This quantity is defined as the normalized change in the probe reflection induced by the pump, Δ R / R 0 ≡( R−R 0 )/ R 0 . Here, R and R 0 are the reflection of the probe with the presence of the pump pulse or without it, respectively. The experimental set-up to measure differential reflection is schematically shown in Supplementary Fig. 7 . The pump and the probe beams are normal incident to the sample and are tightly focused to the sample through a microscope objective lens to spot sizes of 1–2 μm. The reflected probe is collimated by the same lens and is measured by one silicon photodetector as a part of a balanced detector. A set of filters is used to prevent the reflected pump beam from reaching the detector. Before entering the objective lens, a portion of the probe beam is taken as a reference beam, which is sent to the other photodetector of the balanced detector. The power of this reference is carefully adjusted to match the power of the reflected probe with the pump beam blocked, so that the balanced detector has a zero output voltage. With the pump, the power of the probe is changed and a nonzero output is resulted, which is proportional to the differential reflection. The advantage of this balanced detection is that the common mode noise, mostly the intensity noise of the probe, is equally distributed to the probe and reference beams, and is therefore significantly suppressed. To further reduce the noise, the output of the balanced detector is measured with a lock-in amplifier, with the intensity of the pump beam modulated at ~2 kHz with a mechanical chopper. The differential reflection is measured as a function of the probe delay, defined as the time delay of the probe pulse with respect to the pump pulse. This is achieved by controlling the length of the pump path with a linear motor stage. How to cite this article: He, J. et al. Electron transfer and coupling in graphene–tungsten disulfide van der Waals heterostructures. Nat. Commun. 5:5622 doi: 10.1038/ncomms6622 (2014).